Micropatterned substrates coated with neuronal adhesion molecules for high-content study of synapse formation Studying the roles of different proteins and the mechanisms involved in synaptogenesis is hindered by the complexity and heterogeneity of synapse types, and by the spatial and temporal unpredictability of spontaneous synapse formation. Here we demonstrate a robust and high-content method to induce selectively presynaptic or postsynaptic structures at controlled locations. Neurons are cultured on micropatterned substrates comprising arrays of micron-scale dots coated with various synaptogenic adhesion molecules. When plated on neurexin-1β-coated micropatterns, neurons expressing neuroligin-1 exhibit specific dendritic organization and selective recruitment of the postsynaptic scaffolding molecule PSD-95. Furthermore, functional AMPA receptors are trapped at neurexin-1β dots, as revealed by live-imaging experiments. In contrast, neurons plated on SynCAM1-coated substrates exhibit strongly patterned axons and selectively assemble functional presynapses. N-cadherin coating, however, is not able to elicit synapses, indicating the specificity of our system. This method opens the way to both fundamental and therapeutic studies of various synaptic systems. The assembly of the myriad of synapses between neurons during development of the central nervous system represents a pivotal process, which determines the generation, maintenance and function of neural circuitries. At the level of individual axon/dendrite contacts, synaptogenesis is a complex multi-step process initiated by specific adhesion proteins and followed by the recruitment of scaffold molecules and functional receptors [1] , [2] . Several adhesion molecules have been implicated in these processes, including ephrins, cadherins, neurexins (Nrxs), neuroligins (Nlgs), SynCAMs and leucine-rich repeat transmembrane molecules (LRRTMs) [3] , [4] , [5] . Studying the respective roles of these different proteins and the dynamics of the mechanisms involved in synaptogenesis is highly hindered by the complexity and heterogeneity of synapse types, and by the spatial and temporal unpredictability of spontaneous synapse formation. Thus, the development of simplified experimental systems is highly needed to isolate the role of specific adhesion molecules in synapse assembly for both fundamental and therapeutic approaches. Among adhesion molecules, Nrxs and Nlgs are critically involved in synapse formation, differentiation and validation [4] , [6] . Moreover, pathological mutations in their genes are related to autism, X-linked mental retardation and schizophrenia in humans [5] . Nrxs and Nlgs bind to each other through high-affinity recognition between their ectodomains [7] , thus forming a bridge between pre- and postsynaptic membranes, and serving as synaptic organizing complex via intracellular interactions. At the presynaptic level, Nrxs bind the multimodal scaffolding protein CASK and are involved in presynaptic function [4] . At the postsynaptic level, Nlgs bind molecules, including PSD-95 or gephyrin [8] , [9] , serving as scaffolds for the recruitment of glutamate and GABA (γ-aminobutyric acid) receptors, respectively [9] , [10] , [11] , [12] . Importantly, in biomimetic systems like co-cultures or microspheres, Nlgs and Nxrs have the ability to elicit functional pre- and postsynapses, respectively, in contacting primary neurons [10] , [11] , [12] , [13] , [14] , [15] . Furthermore, overexpressing Nlgs in cultured neurons increases the number and size of synapses, whereas downregulation of Nlgs reduces synapse numbers [16] , [17] , [18] , [19] . Besides Nrxs and Nlgs, SynCAMs represent another family of synaptic organizers. SynCAMs are immunoglobulin cell adhesion molecules that are able to form both homophilic and heterophilic interactions, and connect intracellularly with PDZ and FERM domain-containing proteins [20] , [21] , [22] , [23] , [24] . The ability of SynCAMs to trigger synaptic specialization was demonstrated using both knock-out mice and cell culture assays [20] , [21] , [22] , [23] , [24] . Given the diversity in the families, isoforms and splice variants of adhesion molecules potentially implicated in synapse formation, a system allowing high-content screening of synapse formation and function by triggering interaction between specific adhesion molecules would be a valuable tool. The existing biomimetic assays, including beads and co-cultures, are not optimal for such purposes, because of the random distribution of hemisynapses and contamination by endogenous synapses between neurons. To overcome these difficulties, we developed a robust method to spatially control synaptic differentiation, by culturing neurons on micropatterned substrates comprising arrays of individual micron-scale dots coated with N-cadherin, SynCAM1 or Nrx1β, proteins that triggered neuronal development and selective differentiation of functional excitatory pre- or postsynapses, respectively. Considering the simple coating protocol, this assay can be adapted to a wide range of other neuronal adhesion proteins, thus opening the way to the targeted and selective study of the mechanisms underlying synapse formation with unprecedented spatial resolution and statistical production. Moreover, because of its simple design, it can be used with various microscopy techniques and for screening of pharmaceutical compounds modulating synaptogenesis. Neuronal growth on Nrx1β-coated micropatterned substrates To allow the precise formation of hemisynapses at regular locations, we cultured primary hippocampal neurons on specifically designed micropatterned substrates containing a hexagonal array of chemically activated dots (1.5 μm in diameter, separated by 5 μm), surrounded by a non-adhesive background ( Fig. 1a,b ). In a first series of experiments, the dots were specifically coated with recombinant Fc-tagged Nrx1β (Nrx1β-Fc). Nrx1β adsorption was made via Cy5-labelled anti-Fc secondary antibodies, allowing both proper orientation of the adhesive ectodomain and fluorescent visualization of micropatterns. Neurons plated on Nrx1β-coated micropatterned substrates underwent similar developmental stages as described for regular hippocampal cultures grown on homogenously coated glass coverslips coated with Poly-L-Lysine (PLL) [25] ( Supplementary Fig. S1 ). These results indicated that this array of proteins over a cytophobic background did not alter the growth of neurons, in comparison with continuous surfaces classically used for neuronal cultures. 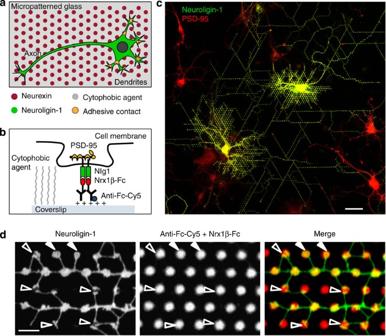Figure 1: Growth and differentiation of neurons cultured on Nrx1β-coated micropatterned substrates. (a) Schematic top view of a neuron growing on Nrx1β-coated micropatterns. Dissociated rat hippocampal neurons (green) were plated on substrates containing a hexagonal array of adhesive dots (1.5 μm) (red) surrounded by a cytophobic agent (grey). Dots were coated with Cy5-conjugated anti-human-Fc antibodies, and either Nrx1β-Fc or human-Fc as a control. (b) Magnified side view of the molecular interactions at a single Nlg1/Nrx1β contact, leading to the recruitment of post-synaptic proteins, including PSD-95 (yellow). (c) Mosaic image of neurons cultured on Nrx1β-Fc-coated micropatterned substrates, transfected with Nlg1-HA, and double immunostained for anti-HA (green) and endogenous PSD-95 (red) at 8 DIV. Note that neurons expressing Nlg1 (yellow) display a strikingly patterned neurite network resembling a subway map compared with that of non-transfected neurons, which have more random morphology (red). The mosaic image was reconstructed from 24 individual high-resolution images. Scale bar, 40 μm. (d) Higher magnification images of a part of a neuron overexpressing Nlg1, highlighting the patterned growth of the dendritic network induced by Nrx1β-Fc-coated dots. Empty and solid arrowheads point to developing and already formed dendritic spine-like structures, respectively, localized at the Nrx1β dots. Scale bar, 5 μm. Figure 1: Growth and differentiation of neurons cultured on Nrx1β-coated micropatterned substrates. ( a ) Schematic top view of a neuron growing on Nrx1β-coated micropatterns. Dissociated rat hippocampal neurons (green) were plated on substrates containing a hexagonal array of adhesive dots (1.5 μm) (red) surrounded by a cytophobic agent (grey). Dots were coated with Cy5-conjugated anti-human-Fc antibodies, and either Nrx1β-Fc or human-Fc as a control. ( b ) Magnified side view of the molecular interactions at a single Nlg1/Nrx1β contact, leading to the recruitment of post-synaptic proteins, including PSD-95 (yellow). ( c ) Mosaic image of neurons cultured on Nrx1β-Fc-coated micropatterned substrates, transfected with Nlg1-HA, and double immunostained for anti-HA (green) and endogenous PSD-95 (red) at 8 DIV. Note that neurons expressing Nlg1 (yellow) display a strikingly patterned neurite network resembling a subway map compared with that of non-transfected neurons, which have more random morphology (red). The mosaic image was reconstructed from 24 individual high-resolution images. Scale bar, 40 μm. ( d ) Higher magnification images of a part of a neuron overexpressing Nlg1, highlighting the patterned growth of the dendritic network induced by Nrx1β-Fc-coated dots. Empty and solid arrowheads point to developing and already formed dendritic spine-like structures, respectively, localized at the Nrx1β dots. Scale bar, 5 μm. Full size image Neurons were transfected with HA-tagged Nlg1, or enhanced green fluorescent protein (EGFP) as a control, 3 days after plating and were allowed to grow for up to 10 days. Cells were either fixed and immunofluorescently stained for Nlg1, PSD-95, or AMPA (alpha-amino-3-hydroxy-5-methyl-4-isoxazolepropionate) receptors (AMPARs), or alternatively used in live-imaging assays. Neurons expressing Nlg1 exhibited strikingly patterned arborizations in comparison with non-transfected cells, reflecting specific recognition between immobilized Nrx1β-Fc and Nlg1 present at the neuronal membrane ( Fig. 1c ). Specifically, the growth of neurites was guided by the topology of the patterns, the overall organization looking like a subway map. Dendrites of neurons expressing Nlg1 grew preferentially along the lines of the Nrx1β-Fc-coated dots and invaded them to a much higher extent than axons ( Supplementary Fig. S2a–c ), consistent with Nlg1 being mainly expressed in the somato-dendritic compartment. As a control, neurons plated on micropatterned substrates coated with human Fc did not develop as well as on Nrx1β-Fc-coated substrates, and the dendritic patterning was not observed even in Nlg1-expressing neurons, revealing specificity of the ligand ( Supplementary Fig. S2f ). The patterning effect was also less obvious in EGFP-expressing neurons grown on Nrx1β-Fc-coated micropatterns ( Supplementary Fig. S2d–f ), indicating that endogenous Nlg1 levels did not accommodate for the large excess of exogenous Nrx1β ligands on micropatterns. When looking at higher magnification, we often observed structures resembling dendritic spines, with a neck originating from dendritic shafts and a head making specific contacts with neighbouring Nrx1β-Fc-coated dots, eventually allowing branching between dendrites ( Fig. 1d ). Thus, by perfectly controlling the adhesive reactivity of the micropatterns, this system induces a directed spreading of the dendritic arbour and selective morphological differentiation of dendrites, mimicking native synaptic structures. Specific induction of excitatory postsynaptic assembly To determine whether this system could further elicit excitatory postsynapse assembly, we examined the accumulation of the postsynaptic proteins Nlg1 and PSD-95 at micropatterns ( Fig. 2 and Supplementary Fig. S3 ). We calculated an enrichment index for PSD-95 and Nlg1 by using immunofluorescence images, and compared the level of enrichment in the presence of the Nrx1β-Fc/Nlg1 interaction and in control conditions, where one of the partners was omitted. Nlg1 and PSD-95:EGFP, as well as endogenous PSD-95, were significantly recruited at dots coated with Nrx1β-Fc ( Fig. 2a,c–e ). As neurons were plated at low density and observed at relatively young stages (8–9 days in vitro (DIV)), endogenous synapses were scarce and rarely localized at Nrx1β-Fc-coated dots ( Supplementary Fig. S4 ); thus, we could neglect their contribution to postsynaptic differentiation induced by Nrx1β-Fc. As controls, neither PSD-95 nor EGFP were recruited at Nrx1β-Fc-coated dots in the absence of Nlg1 expression ( Fig. 2b–e ), and neither Nlg1 nor PSD-95 were recruited at Fc-coated micropatterns ( Fig. 2c–e ), demonstrating the specificity of the Nrx1β/Nlg1 interaction in this assay. Importantly, as each neuron was spreading over hundreds of individual dots, we quickly reached very high statistics ( Fig. 2e ). Taken together, these data indicate that neuronal contacts formed at Nrx1β-coated micropatterns selectively assemble major proteins involved in excitatory postsynaptic differentiation, independently of native synapses. 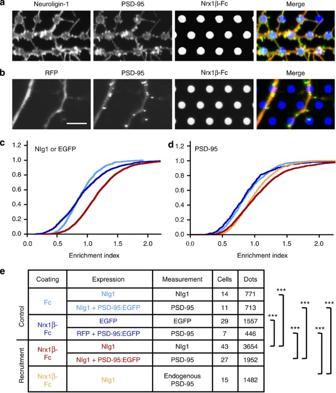Figure 2: Quantification of post-synaptic protein recruitment at Nrx1β-coated micropatterns. (a) Dendritic part of a neuron transfected with Nlg1-HA and PSD-95:EGFP, showing the enrichment of Nlg1 (red) and PSD-95 (green) at Nrx1β-Fc-coated dots (blue). (b) Dendritic part of a neuron transfected with red fluorescent protein (RFP) and PSD-95:EGFP, showing the lack of recruitment of RFP (red) and PSD-95 (green) at Nrx1β-Fc-coated dots (blue). Scale bar, 5 μm. (c,d) Cumulative distributions of the enrichment index of Nlg1 and EGFP (c), or PSD-95 (d), in the different conditions detailed in the table below. The enrichment index was calculated at individual dots by dividing the average fluorescence intensity of the given protein within the area of the dendrite colocalizing with coated dots, by the average fluorescence intensity of dendritic parts located between the patterns. (e) The table contains the different conditions and the number of cells, and dots used for quantification. Data sets were collected from three different neuronal cultures and compared using a two-way analysis of variance followed by Bonferroni’s parametric post test (***P<0.001). The two control conditions (in blue) were not statistically different. Figure 2: Quantification of post-synaptic protein recruitment at Nrx1β-coated micropatterns. ( a ) Dendritic part of a neuron transfected with Nlg1-HA and PSD-95:EGFP, showing the enrichment of Nlg1 (red) and PSD-95 (green) at Nrx1β-Fc-coated dots (blue). ( b ) Dendritic part of a neuron transfected with red fluorescent protein (RFP) and PSD-95:EGFP, showing the lack of recruitment of RFP (red) and PSD-95 (green) at Nrx1β-Fc-coated dots (blue). Scale bar, 5 μm. ( c , d ) Cumulative distributions of the enrichment index of Nlg1 and EGFP ( c ), or PSD-95 ( d ), in the different conditions detailed in the table below. The enrichment index was calculated at individual dots by dividing the average fluorescence intensity of the given protein within the area of the dendrite colocalizing with coated dots, by the average fluorescence intensity of dendritic parts located between the patterns. ( e ) The table contains the different conditions and the number of cells, and dots used for quantification. Data sets were collected from three different neuronal cultures and compared using a two-way analysis of variance followed by Bonferroni’s parametric post test (*** P <0.001). The two control conditions (in blue) were not statistically different. Full size image Contact formation between filopodia and Nrx1β-coated dots To gain insight into the dynamics of postsynapse formation, we combined this system with long-term live-cell imaging. Neurons plated on Nrx1β-Fc-coated substrates were cotransfected with Nlg1 and PSD-95:EGFP, and were monitored at DIV 6 for several hours. By focusing on freely moving dendritic filopodia in relation to the surrounding dots, we observed that filopodia often contained a leader PSD-95 cluster, reaching out to Nrx1β-Fc micropatterns and establishing firm contact within hours ( Fig. 3a and Supplementary Movie 1 ). These mobile precursor complexes containing Nlg1 and PSD-95 are likely to serve as preformed postsynaptic hotspots for establishment of new functional excitatory synapses [26] , [27] . 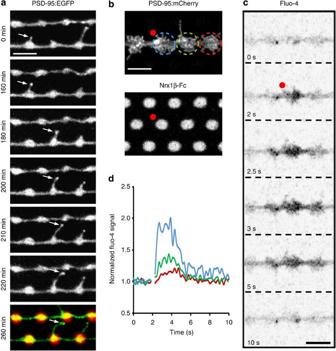Figure 3: Synapse dynamics and function observed on Nrx1β-coated micropatterns. (a) Image series showing Nrx1β/Nlg1 contact formation in neurons transfected with Nlg1 and PSD-95:EGFP. Note the presence of pre-assembled PSD-95:EGFP clusters at the tips of dendritic filopodia (arrow), which eventually become the sites of primary contacts with Nrx1β-Fc-coated dots. The specific contacts persisted for at least 50 min after initial adhesion. The merged image showing PSD-95:EGFP (green) and Nrx1β-Fc-coated dots (red) was taken at the end of the experiment. Scale bar, 5 μm. (b–d) Neurons transfected with Nlg1-HA and PSD-95:mCherry were loaded with Fluo-4 and the changes in intracellular calcium level evoked by MNI-glu uncaging was monitored. (b) Image of a dendritic segment, highlighting PSD-95:mCherry accumulation at Nrx1β-Fc-coated dots. The bi-photon laser pulse used to trigger glutamate uncaging was positioned close to a micropattern (red dot). (c) Corresponding time sequence of the Fluo-4 signal upon glutamate uncaging. Note that the calcium signal starts to increase right after glutamate uncaging, specifically at the dot in closest proximity to the laser position. The signal then propagates to the neighbouring dots and progressively decreases. Scale bar, 5 μm. (d) The graph shows different calcium transient responses, normalized to the baseline level, measured either at the location of uncaging (blue), or at neighbouring patterns located closer to (green) or further from (red) the uncaging spot, as indicated inb. Figure 3: Synapse dynamics and function observed on Nrx1β-coated micropatterns. ( a ) Image series showing Nrx1β/Nlg1 contact formation in neurons transfected with Nlg1 and PSD-95:EGFP. Note the presence of pre-assembled PSD-95:EGFP clusters at the tips of dendritic filopodia (arrow), which eventually become the sites of primary contacts with Nrx1β-Fc-coated dots. The specific contacts persisted for at least 50 min after initial adhesion. The merged image showing PSD-95:EGFP (green) and Nrx1β-Fc-coated dots (red) was taken at the end of the experiment. Scale bar, 5 μm. ( b – d ) Neurons transfected with Nlg1-HA and PSD-95:mCherry were loaded with Fluo-4 and the changes in intracellular calcium level evoked by MNI-glu uncaging was monitored. ( b ) Image of a dendritic segment, highlighting PSD-95:mCherry accumulation at Nrx1β-Fc-coated dots. The bi-photon laser pulse used to trigger glutamate uncaging was positioned close to a micropattern (red dot). ( c ) Corresponding time sequence of the Fluo-4 signal upon glutamate uncaging. Note that the calcium signal starts to increase right after glutamate uncaging, specifically at the dot in closest proximity to the laser position. The signal then propagates to the neighbouring dots and progressively decreases. Scale bar, 5 μm. ( d ) The graph shows different calcium transient responses, normalized to the baseline level, measured either at the location of uncaging (blue), or at neighbouring patterns located closer to (green) or further from (red) the uncaging spot, as indicated in b . Full size image Functional glutamate receptor recruitment at Nrx1β adhesions To examine whether PSD-95 scaffolds assembled at Nrx1β-Fc-coated dots were recruiting functional glutamate receptors, we used bi-photon glutamate uncaging and calcium imaging. Neurons were cotransfected with Nlg1 and PSD-95:mCherry to monitor postsynaptic differentiation in live conditions and were incubated with the cell-permeant calcium indicator Fluo-4 ( Fig. 3b,c ). When 4-methoxy-7-nitroindolinyl-caged L-glutamate (MNI-glu) was uncaged in the vicinity of dendritic segments, showing accumulation of PSD-95:mCherry at Nrx1β-Fc dots, local and selective calcium transients were recorded ( Fig. 3c,d and Supplementary Movie 2 ), revealing the presence of functional glutamate receptors. The increase in calcium signal upon glutamate uncaging at Nrx1β-Fc dots was 67±8% ( n =12 cells), identical to the responses obtained in 3-week-old neurons at endogenous synapses (69±9%, 30 cells), further indicating that molecular complexes assembled at Nrx1β micropatterns resemble native postsynapses. In a previous study using glutamate uncaging at Nrx1β-coated beads, we showed that such calcium transients are due to voltage-gated calcium channels, which open upon membrane depolarization induced by AMPAR activation [12] . Thus, it is likely that the glutamate receptors recruited at Nrx1β-coated micropatterns contain AMPARs. Trapping of surface diffusing AMPARs at Nrx1β adhesions To directly demonstrate the recruitment of AMPARs at Nrx1β-induced postsynaptic structures, we immunolabelled AMPARs in neurons expressing Nlg1. Using a monoclonal anti-GluA2 antibody for live labelling, we demonstrated that endogenous surface AMPARs were recruited at Nrx1β dots, and were clearly colocalized with PSD-95 ( Fig. 4a ). It was previously shown that AMPARs are anchored at the postsynaptic density via specific interactions with scaffolding molecules, such as PSD-95, but they also undergo dynamic exchange between synaptic and extra-synaptic membrane compartments [15] , [28] , [29] . To gain insight into the dynamics of AMPARs recruited at Nrx1β-induced postsynaptic structures, we followed the mobility of individual AMPARs in neurons expressing Nlg1 and grown on micropatterned substrates coated with Nrx1β or Fc ( Fig. 4b,c ). Surface AMPARs were sparsely labelled by adding anti-GluA2 antibodies conjugated to Atto647N dyes in the observing solution, and two-dimensional trajectories were recorded using a single-molecule tracking technique 30 . Importantly, oblique laser illumination allowed the detection of single dye fluorescence in focal planes close to the substrate where Nrx1β/Nlg1 adhesions are localized. We calculated the distribution of instantaneous diffusion coefficients ( D ) of AMPAR trajectories localized on the patterns, and trajectories localized on dendritic parts lying between patterns, for both types of coatings ( Fig. 4d,e ). In all conditions, the distributions contained two well-separated populations, a fast-diffusing one ( D >0.01 μm 2 s −1 ) and a slow-diffusing one ( D <0.01 μm 2 s −1 ). The proportion of fast-moving AMPARs was significantly reduced at Nrx1–Fc patterns compared with the Fc coating, where it remained as high as outside patterns ( Fig. 4d,e ), revealing that AMPARs get selectively confined at Nrx1β/Nlg1 contacts. These results indicate that Nrx1β-induced adhesions are capable of trapping surface diffusing AMPARs, similar to native synapses [15] , [28] . 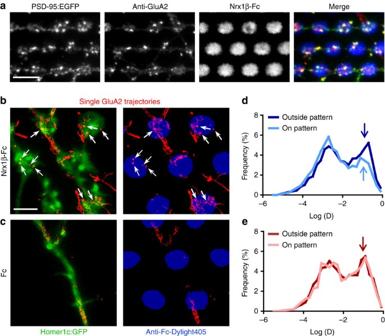Figure 4: Single-molecule tracking of surface AMPARs in neurons cultured on Nrx1β-coated micropatterned substrates. (a) Dendritic segments of a neuron transfected with Nlg1-HA and PSD-95:GFP, where endogenous AMPARs at the cell surface were live labelled with anti-GluA2 antibodies. Note the AMPAR accumulation at Nrx1β-coated micropatterns and the clear colocalization with PSD-95 (arrows). Scale bar, 5 μm. (b,c) The surface diffusion of endogenous AMPARs was monitored by tracking individual anti-GluA2 antibodies conjugated to Atto-647 dyes (red traces), in neurons cotransfected with Nlg1-HA and Homer1c:GFP, and grown for 8 DIV on micropatterned substrates coated with either Nrx1β-Fc (b) or Fc (c). Note AMPAR confinement at Nrx1β-coated dots, partially colocalizing with Homer1c:GFP puncta (arrows). Scale bar, 2 μm. (d,e) The graphs show the distributions of the instantaneous diffusion coefficients of individual AMPAR trajectories, calculated and plotted on a logarithmic scale, for neurons grown on micro-patterned substrates coated with Nrx1β-Fc (d) or Fc (e). The trajectories were distinguished according to whether they were localized inside or outside micropatterns. Note a significant drop of the more mobile AMPARs (blue arrows), owing to AMPAR trapping at Nrx1β-induced adhesions, which was not observed in the Fc condition (red arrow). Distributions were calculated from 2,000 to 3,000 individual trajectories from 8 cells for Nrx1β-Fc-coated substrates and 6 cells for Fc-coated substrates. The mobile AMPAR fractions inside and outside Nrx1β-coated micropatterns were 25±2% (mean±s.e.m., seven regions) and 33±2% (six regions), respectively (P=0.005 by unpaired Student’st-test). The mobile AMPAR fractions inside and outside Fc-coated micropatterns were 39±4% (mean±s.e.m., seven regions) and 36±4% (six regions), respectively (not significant). The mobile AMPAR fraction on Nrx1β was significantly lower than on Fc-coated dots (P<0.005). Figure 4: Single-molecule tracking of surface AMPARs in neurons cultured on Nrx1β-coated micropatterned substrates. ( a ) Dendritic segments of a neuron transfected with Nlg1-HA and PSD-95:GFP, where endogenous AMPARs at the cell surface were live labelled with anti-GluA2 antibodies. Note the AMPAR accumulation at Nrx1β-coated micropatterns and the clear colocalization with PSD-95 (arrows). Scale bar, 5 μm. ( b , c ) The surface diffusion of endogenous AMPARs was monitored by tracking individual anti-GluA2 antibodies conjugated to Atto-647 dyes (red traces), in neurons cotransfected with Nlg1-HA and Homer1c:GFP, and grown for 8 DIV on micropatterned substrates coated with either Nrx1β-Fc ( b ) or Fc ( c ). Note AMPAR confinement at Nrx1β-coated dots, partially colocalizing with Homer1c:GFP puncta (arrows). Scale bar, 2 μm. ( d , e ) The graphs show the distributions of the instantaneous diffusion coefficients of individual AMPAR trajectories, calculated and plotted on a logarithmic scale, for neurons grown on micro-patterned substrates coated with Nrx1β-Fc ( d ) or Fc ( e ). The trajectories were distinguished according to whether they were localized inside or outside micropatterns. Note a significant drop of the more mobile AMPARs (blue arrows), owing to AMPAR trapping at Nrx1β-induced adhesions, which was not observed in the Fc condition (red arrow). Distributions were calculated from 2,000 to 3,000 individual trajectories from 8 cells for Nrx1β-Fc-coated substrates and 6 cells for Fc-coated substrates. The mobile AMPAR fractions inside and outside Nrx1β-coated micropatterns were 25±2% (mean±s.e.m., seven regions) and 33±2% (six regions), respectively ( P =0.005 by unpaired Student’s t -test). The mobile AMPAR fractions inside and outside Fc-coated micropatterns were 39±4% (mean±s.e.m., seven regions) and 36±4% (six regions), respectively (not significant). The mobile AMPAR fraction on Nrx1β was significantly lower than on Fc-coated dots ( P <0.005). Full size image Induction of functional presynapses on SynCAM1 substrates After having thoroughly characterized the properties of Nrx1β-coated micropatterns on postsynaptic induction, we asked whether the design could be reversed to elicit selective presynaptic differentiation in axons. We first tried to culture neurons on substrates coated with purified Nlg1-6His, immobilized on the micropatterns through an anti-6His antibody ( Supplementary Fig. S5a,b ). We verified by anti-Fc immunostaining that purified Nrx1β-Fc bound specifically to the Nlg1-coated dots, indicating intact adhesive function of Nlg1-6His ( Supplementary Fig. S5c ). Surprisingly, neurons had difficulties to grow on Nlg1-coated substrates and were very sensitive to further treatments, such as immunostaining. Moreover, when we were able to keep the neurons for 10 DIV on Nlg1-coated micropatterned substrates, neither axons nor dendrites were particularly patterned ( Supplementary Fig. S5d ), and axons did not strongly accumulate the presynaptic marker synapsin, even in neurons expressing Nrx1β-HA ( Supplementary Fig. S5e ). Thus, in contrast with previously reported effects in co-culture and bead assays [13] , [14] , Nlg1 immobilized on micropatterns did not induce robust presynaptic differentiation. To examine whether our system could be used to induce presynapses using synaptogenic proteins other than Nlg1, we cultured neurons on micropatterned substrates coated with SynCAM1, an adhesion molecule involved in axonal growth and synaptic differentiation [20] , [22] , [24] ( Fig. 5a,b ). Neurons cultured on SynCAM1-Fc-coated micropatterns grew very well and extended both axons and dendrites, without the need of overexpressing SynCAM1 ( Fig. 5c ). Neurons accumulated endogenous SynCAM1 on the dots, reflecting strong homophilic SynCAM1/SynCAM1 interactions ( Fig. 5c,d ). Strikingly, axons were highly patterned and showed synapsin accumulation at SynCAM1-coated dots, indicating presynaptic differentiation ( Fig. 5d ). In contrast, dendrites growing on SynCAM1-coated micropatterned substrates were less affected and did not particularly accumulate PSD-95 at SynCAM1-coated dots ( Fig. 5c,e ). 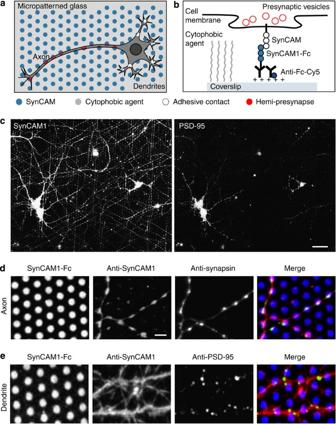Figure 5: Neuronal growth and differentiation on SynCAM1-coated micropatterned substrates. (a) Schematic top view of a neuron growing on SynCAM1-Fc-coated micropatterns (blue). Because of the homophilic interaction of SynCAMs, adhesive contacts (dashed outline) are expected on both axon and dendrites. Expected location of induced presynapse formation is marked in dark red. (b) Magnified side view of the interaction at a single SynCAM1/SynCAM contact, leading to the recruitment of presynaptic vesicles (red). (c) Mosaic image of neurons cultured for 7 DIV on micropatterned substrates coated with SynCAM1-Fc. The cells were dual labelled for endogenous SynCAM1 and PSD-95. Note the specific axonal growth along micropatterns and the random growth of dendrites. Scale bar, 30 μm. (d,e) High-magnification images of DIV 7 neurons dual labelled either for endogenous SynCAM1 and synapsin, or for SynCAM1 and PSD-95, respectively. (d) Axonal segment showing specific accumulation of both SynCAM1 and synapsin at contact sites with SynCAM1-Fc-coated micropatterns. Scale bar, 5 μm. (e) Image of a dendritic segment showing that PSD-95 accumulation was randomly distributed. Figure 5: Neuronal growth and differentiation on SynCAM1-coated micropatterned substrates. ( a ) Schematic top view of a neuron growing on SynCAM1-Fc-coated micropatterns (blue). Because of the homophilic interaction of SynCAMs, adhesive contacts (dashed outline) are expected on both axon and dendrites. Expected location of induced presynapse formation is marked in dark red. ( b ) Magnified side view of the interaction at a single SynCAM1/SynCAM contact, leading to the recruitment of presynaptic vesicles (red). ( c ) Mosaic image of neurons cultured for 7 DIV on micropatterned substrates coated with SynCAM1-Fc. The cells were dual labelled for endogenous SynCAM1 and PSD-95. Note the specific axonal growth along micropatterns and the random growth of dendrites. Scale bar, 30 μm. ( d , e ) High-magnification images of DIV 7 neurons dual labelled either for endogenous SynCAM1 and synapsin, or for SynCAM1 and PSD-95, respectively. ( d ) Axonal segment showing specific accumulation of both SynCAM1 and synapsin at contact sites with SynCAM1-Fc-coated micropatterns. Scale bar, 5 μm. ( e ) Image of a dendritic segment showing that PSD-95 accumulation was randomly distributed. Full size image To show whether the hemisynapses formed on SynCAM-1-coated dots were functional, neurons were live-labelled with an antibody against the luminal domain of synaptotagmin. Strong synaptotagmin staining was observed at axonal processes in contact with SynCAM1-Fc-coated dots ( Fig. 6a ), indicating antibody uptake and, thereby, the presence of actively recycling presynapses. Quantification of the levels of overlap between synaptic puncta and micropatterns ( Supplementary Fig. S6 ) revealed a significant enrichment of both synapsin and synaptotagmin puncta at SynCAM1-coated dots, compared with PSD-95 or the control value expected from a random distribution of puncta ( Fig. 6b ). 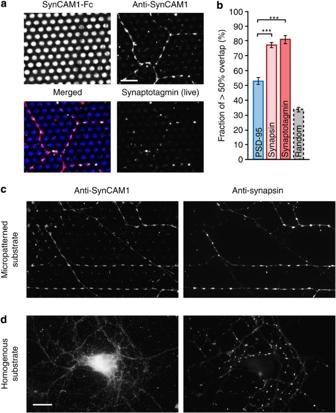Figure 6: Formation of functional presynapses on SynCAM1-coated micropatterned substrates. (a) Axonal segments of a neuron cultured for 7 DIV on micropatterned substrates coated with SynCAM1-Fc. Cells were live labelled with Oyster550-conjugated antisynaptotagmin luminal domain, followed by fixation and immunostaining for endogenous SynCAM1. Note the strong accumulation of both SynCAM1 and synaptotagmin at the dots, revealing the presence of actively recycling presynapses. Scale bar, 10 μm. (b) Neurons at DIV 7 were growing on micropatterned substrates coated with SynCAM1-Fc and either fixed and immunostained for synapsin, or fixed after live incubation with Oyster550-conjugated antisynaptotagmin luminal domain). The graph shows the percentage of synapsin or synaptotagmin puncta having more than 50% overlapping area with the micropatterns (average per cell±s.e.m.). Data were collected from three different neuronal cultures (synapsin: 39 cells, 4,121 puncta; PSD-95: 33 cells, 3,438 puncta; synaptotagmin: 5 cells, 233 puncta) and were compared using a one-way analysis of variance followed by Bonferroni’s parametric post test (***P<0.001). The grey bar indicates the value for a random distribution of puncta calculated from the percentage of area occupied by dots on the substrate (mean±s.e.m.,n=27 regions). (c,d) Images of neurons cultured for 7 DIV either on micropatterned substrates coated with SynCAM1-Fc or on coverslips homogenously coated with SynCAM1-Fc, respectively, and dual labelled for endogenous SynCAM1 and synapsin. Note the random versus patterned distribution of synapses on the homogenous and micropatterned substrate, respectively. Scale bar, 10 μm. Figure 6: Formation of functional presynapses on SynCAM1-coated micropatterned substrates. ( a ) Axonal segments of a neuron cultured for 7 DIV on micropatterned substrates coated with SynCAM1-Fc. Cells were live labelled with Oyster550-conjugated antisynaptotagmin luminal domain, followed by fixation and immunostaining for endogenous SynCAM1. Note the strong accumulation of both SynCAM1 and synaptotagmin at the dots, revealing the presence of actively recycling presynapses. Scale bar, 10 μm. ( b ) Neurons at DIV 7 were growing on micropatterned substrates coated with SynCAM1-Fc and either fixed and immunostained for synapsin, or fixed after live incubation with Oyster550-conjugated antisynaptotagmin luminal domain). The graph shows the percentage of synapsin or synaptotagmin puncta having more than 50% overlapping area with the micropatterns (average per cell±s.e.m.). Data were collected from three different neuronal cultures (synapsin: 39 cells, 4,121 puncta; PSD-95: 33 cells, 3,438 puncta; synaptotagmin: 5 cells, 233 puncta) and were compared using a one-way analysis of variance followed by Bonferroni’s parametric post test (*** P <0.001). The grey bar indicates the value for a random distribution of puncta calculated from the percentage of area occupied by dots on the substrate (mean±s.e.m., n =27 regions). ( c , d ) Images of neurons cultured for 7 DIV either on micropatterned substrates coated with SynCAM1-Fc or on coverslips homogenously coated with SynCAM1-Fc, respectively, and dual labelled for endogenous SynCAM1 and synapsin. Note the random versus patterned distribution of synapses on the homogenous and micropatterned substrate, respectively. Scale bar, 10 μm. Full size image To compare synapse formation on micropatterned substrates versus classical substrates, we also plated neurons on glass substrates homogeneously coated with SynCAM1. In these conditions, neurons grew well, showed disorganized neurite networks and formed synapses at random locations ( Fig. 6c,d ). Furthermore, it was difficult to assess whether synapsin puncta reflected hemisynapses formed with SynCAM1 ligands immobilized on the substrate, or actual synapses formed between axons and dendrites. Thus, SynCAM1-coated micropatterned substrates are highly efficient to induce functional presynapses in a spatially controlled manner, thus overcoming limitations of the homogeneously coated substrates. No synapse induction on N-cadherin-coated substrates To prove that the induction of pre- and postsynaptic structures in our assay was specific of the adhesion molecule used for coating, we plated neurons on micropatterned substrates coated with N-cadherin-Fc ( Fig. 7a,b ), a non-synaptogenic adhesion molecule rather involved in axonal growth and neurite branching [31] , [32] . Neurons developed faster on those substrates than on micropatterned substrates coated with Nrx1β-Fc or on regular glass coverslips coated with PLL, but to similar rates as on glass coverslips homogeneously coated with N-cadherin-Fc 32 ( Supplementary Fig. S1 ). Similar to SynCAM1, N-cadherin-based adhesion was strong enough to support neuronal growth, and extended patterned arborization of both axons and dendrites in the absence of N-cadherin overexpression ( Fig. 7c,d ). Endogenous N-cadherin accumulated at N-cadherin-coated dots, revealing specific homophilic interactions, but neither synapsin nor PSD-95 accumulated at N-cadherin-coated dots ( Fig. 7c,e ). The lack of synapse induction by N-cadherin in our assay is in agreement with previous studies using co-cultures or N-cadherin-coated beads [11] , [12] , [13] , and is compatible with the dispensable effect of N-cadherin in aligning pre- and postsynapses 33 . 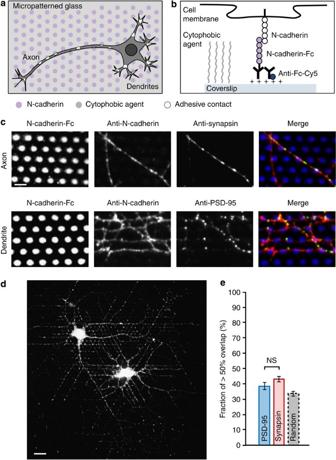Figure 7: Neuronal growth and differentiation on N-cadherin-coated micropatterned substrates. (a) Schematic top view of a neuron growing on N-cadherin-Fc-coated micropatterns (purple). Because of the homophilic interaction of N-cadherins, adhesive contacts (dashed outline) are expected on both axon and dendrites. (b) Magnified side view of the molecular interactions at a single N-cadherin contact. (c) Enlarged images showing axonal and dendritic parts of DIV 7 neurons, which were dual labelled either for endogenous N-cadherin and synapsin, or N-cadherin and PSD-95. Note the enrichment of endogenous N-cadherin in both axon and dendrites at N-cadherin-coated micropatterns, whereas synapsin and PSD-95 were randomly distributed in both axon and dendrites. Scale bar, 5 μm. (d) Image of neurons cultured for 7 DIV on N-cadherin-Fc-coated micro-patterned substrates, immunostained for endogenous N-cadherin. Note the patterned arborization of axons and dendrite branching, reflecting the interaction with the N-cadherin-Fc-coated dots. Scale bar, 20 μm. (e) Graph showing the percentage of synapsin or PSD-95 puncta, showing more than 50% overlapping area with the micropatterns. Quantification was made on neurons (DIV 7) cultured on micropatterned substrates coated either with N-cadherin-Fc and immunostained for synapsin or PSD-95 (synapsin: 8 cells, 1,286 puncta; PSD-95: 16 cells, 3,471 puncta). The data for the two conditions were compared using unpaired Student’st-test (NS: not significant;P=0.44). The grey bar indicates the value for a random distribution of puncta on the substrate (mean±s.e.m.,n=27). Figure 7: Neuronal growth and differentiation on N-cadherin-coated micropatterned substrates. ( a ) Schematic top view of a neuron growing on N-cadherin-Fc-coated micropatterns (purple). Because of the homophilic interaction of N-cadherins, adhesive contacts (dashed outline) are expected on both axon and dendrites. ( b ) Magnified side view of the molecular interactions at a single N-cadherin contact. ( c ) Enlarged images showing axonal and dendritic parts of DIV 7 neurons, which were dual labelled either for endogenous N-cadherin and synapsin, or N-cadherin and PSD-95. Note the enrichment of endogenous N-cadherin in both axon and dendrites at N-cadherin-coated micropatterns, whereas synapsin and PSD-95 were randomly distributed in both axon and dendrites. Scale bar, 5 μm. ( d ) Image of neurons cultured for 7 DIV on N-cadherin-Fc-coated micro-patterned substrates, immunostained for endogenous N-cadherin. Note the patterned arborization of axons and dendrite branching, reflecting the interaction with the N-cadherin-Fc-coated dots. Scale bar, 20 μm. ( e ) Graph showing the percentage of synapsin or PSD-95 puncta, showing more than 50% overlapping area with the micropatterns. Quantification was made on neurons (DIV 7) cultured on micropatterned substrates coated either with N-cadherin-Fc and immunostained for synapsin or PSD-95 (synapsin: 8 cells, 1,286 puncta; PSD-95: 16 cells, 3,471 puncta). The data for the two conditions were compared using unpaired Student’s t -test (NS: not significant; P =0.44). The grey bar indicates the value for a random distribution of puncta on the substrate (mean±s.e.m., n =27). Full size image We developed a robust method to induce targeted and selective formation of hemisynapses with high statistics, by culturing neurons on micropatterned substrates coated with Nrx1β or SynCAM1. For each neuron, this system can trigger hundreds of micron-scale contacts, specifically recruiting major proteins involved in excitatory postsynaptic differentiation (Nlg1, PSD-95 and AMPARs) or presynaptic assembly (SynCAM-1 and synapsin). Our assay can be combined with various imaging techniques, including immunocytochemistry to screen the accumulation of synaptic components, long-term live cell recordings to probe the kinetics of synapse differentiation, local photo-activation to probe functional synaptic properties and high-resolution single-molecule tracking. Substrate adhesion, a key parameter that determines the growth and survival of neurons in vitro , is governed by a number of factors, including the number of ligand molecules presented to the cells, the number of surface receptors expressed by cells, the affinity of ligand/receptor interactions and the area available for these interactions. In this micropattern assay, the area available for cell adhesion is around 38% of the total substrate area, the rest being covered by a cytophobic agent. To balance this reduction in adhesion area, we had to modify the other three factors, namely (1) controlling the number of functional ligand molecules using saturating concentrations of secondary antibodies; (2) enhancing the affinity of ligand/receptor interaction by choosing adhesion molecules with high binding affinity; (3) and/or increasing the number of available receptors by transfection. As a result, we could reproduce normal or enhanced growth of neurons on micropatterned substrates coated with Nrx1β, SynCAM1 and N-cadherin compared with regular homogenously coated substrates. In comparison, coatings of micropatterned substrates with PLL or Fc were not sufficient to support normal neuronal growth. As patterned neurite development and hemisynaptic differentiation on Nrx1β-coated substrates were selective of Nlg1-expressing neurons, Nlg1 localized at the cell surface is likely to be the primary binding partner for Nrx1β immobilized at the dots. Although soluble Nrx1β can bind endogenous Nlg1 at the surface of hippocampal neurons [26] , in our system endogenous Nlg1 levels could not accommodate for the large excess of exogenous Nrx1β ligands on the micropatterns. Thus, overexpression of Nlg1 was required to establish Nrx1β/Nlg1 adhesions restricted to the micron-scale dots, ensuring the isolated study of specific molecular interactions. The reason why Nrx cannot induce postsynapses in the absence of Nlg1 expression maybe that the levels of Nrx receptors, including Nlgs and LRRTMs, in cultured neurons are low compared with that of the receptors for SynCAMs and N-cadherin. Another explanation is that N-cadherin and SynCAM1 (but not Nrx1) can form cis -dimers through extracellular interactions [7] , [34] , [35] , thereby locally increasing their concentration. Nlg1 immobilized on micropatterns was unable to induce robust neuronal growth and reproducible presynaptic differentiation in contrast to what was reported in co-cultures and lipid-coated beads [13] , [14] . There are several potential explanations for this finding: (1) although Nrxs have also been reported in dendrites 36 , those molecules are mostly presynaptic; thus, neuronal adhesion to Nlg1-coated dots is mediated essentially by axons, which may not be sufficient to promote strong somato-dendritic adhesion and cell survival; (2) purified Nlg1 protein may be more fragile than Nrx1β and get degraded throughout several days at 37 °C; (3) Nlg1 can induce presynaptic differentiation only when it is freely diffusible in lipid membranes and not when immobilized on a substrate [14] , [37] , [38] ; and (4) Nlg1, which is assembled as a constitutive dimer through interactions between extracellular AchE-like domains [14] , [39] , does not function properly when presented as a Nlg1-6His monomer. Nevertheless, SynCAM1-coated substrates elicited a very robust patterned axonal arborization and presynaptic differentiation without the need for SynCAM overexpression. Probably, high endogenous SynCAM levels in hippocampal cells and high-affinity binding between SynCAMs [20] , [21] enable such strong neuronal differentiation. Moreover, homophilic adhesion has the advantage of expanding the surface of interaction between micropatterns and neurons to both axons and dendrites. The accumulation of endogenous SynCAM1 at SynCAM1-Fc-coated dots indicated homophilic SynCAM1/SynCAM1 interactions, although interactions with presynaptic SynCAM2 may also occur [21] . In contrast, SynCAM1-Fc on micropatterns did not induce strong postsynaptic differentiation, as already reported with SynCAM1-coated beads 40 or neuronal co-cultures with heterologous cells expressing SynCAM1 (ref. 11 ). One possibility is that SynCAMs lack postsynaptic organizing capability, or have to work in parallel with other synaptic presynaptic cell adhesion molecules to induce a postsynaptic differentiation 41 . Although SynCAM1 was immobilized on micropatterns through antibodies, thus lacking membrane diffusion as in spontaneous contacts, this did not alter its capacity to induce neurite growth and synapse differentiation. Moreover, the use of recombinant SynCAM1-Fc, which can spontaneously dimerize through disulphide bonds in the Fc moiety, may be important to promote SynCAM1 dimerization through extracellular FNIII domains and enhance its function in this assay [35] . Once the specific contacts were generated robustly and reliably, we investigated whether these contacts were able to trigger further processes implicated in pre- and postsynapse assembly. The scaffolding protein PSD-95 is one of the earliest detected proteins at synapses [1] , [2] and can interact directly with the carboxy-terminal PDZ domain binding motif of Nlg1 (ref. 8 ). In addition, PSD-95 was previously shown to be recruited at neuronal contacts with heterologous cells expressing Nrx1β, microbeads coated with purified Nrx1β or antibody cross-linked Nrx1β [10] , [11] , [12] , [15] . In line with these findings, we demonstrated that PSD-95 is enriched at Nrx1β micropatterns, indicating that Nrx1β-Fc/Nlg1 adhesions are able to recruit postsynaptic scaffolding molecules. The recruitment of PSD-95 is likely to involve both directed transport of preformed clusters as indicated by our long-term live cell recordings confirming previous reports [26] , [27] , as well as trapping of diffusible PSD-95 (ref. 15 ). Besides scaffolding molecules, glutamate receptors are also crucial for synaptic function. By using glutamate uncaging and live antibody staining, we further revealed that functional AMPARs were also present at Nrx1β micropatterns. Although earlier reports indicated minor recruitment of AMPARs at Nrx1β-induced adhesions [10] , [11] , we recently showed that AMPARs could be recruited at novel Nrx1β/Nlg1 adhesions in an activity-independent manner, through a mechanism implicating essentially GluA2-containing AMPARs [12] , [15] . To significantly improve the detection of synaptic events specifically associated with Nrx1/Nlg1 adhesion sites at the substrate level, we used oblique illumination in single-molecule tracking experiments and showed that surface-diffusing AMPARs could be specifically trapped at Nrx1β-induced adhesions. Overall, our assay can be used to specifically induce postsynapse assembly by establishing stable and robust Nrx1β/Nlg1 contacts at spatially controlled locations, triggering the recruitment of scaffolding molecules and functional AMPARs, similar to what was described at native synapses [15] , [28] . A recent study using neurons expressing pHluorin-tagged AMPAR subunits and plated on substrates uniformly coated with Nrx1β demonstrated local exocytic events close to Nrx1β/Nlg1 contact sites, upon neuronal stimulation 42 . To unify those observations, we propose a two-step model where AMPAR, which are exocytosed extrasynaptically can subsequently diffuse laterally and get trapped at synapses by PSD scaffolds assembled by Nrx/Nlg adhesions 43 . On SynCAM1-coated patterns, we demonstrated the differentiation of functional presynapses through the accumulation of endogenous SynCAM1, synapsin and actively recycling synaptotagmin. Given the large proportion of glutamatergic neurons in hippocampal cultures, and the tendency for SynCAM1 to induce more excitatory versus inhibitory synapses in co-culture assays and in transfected neurons [21] , [41] , it is likely that most presynapses formed on SynCAM1-Fc-coated micropatterns represent glutamatergic terminals. Given the strong presynaptic differentiation induced by SynCAM1-coated micropatterns, the combination of this assay with total internal reflection fluorescence microscopy may represent a promising tool for high-resolution study of the mechanisms of vesicular release at the presynapse. The difficulty to study the process of synapse formation has led to the development of several biomimetic tools based on synaptogenic adhesion molecules, including co-cultures [10] , [11] , [13] , [20] , microspheres [10] , [12] , [14] and protein clusters [9] , [15] , [27] . All these tools aim to trigger synaptogenesis in a more controlled way compared with regular neuronal cultures, where spontaneous axon/dendrite contacts form unpredictably [1] , [2] . The strong advantage of micropatterned substrates over such experiments is that one precisely controls the position where to expect synapse formation. Patterned substrates with large adhesive islands and/or thin lines were previously used to generate autapses, induce axonal elongation and growth cone migration, or build simplified neuronal networks [44] , [45] , [46] , [47] , [48] , but not to locally induce synaptogenesis with specific neuronal adhesion molecules, as described here. A ‘synapse microarray’ was recently reported to enable high-throughput screening, using non-neuronal cells expressing Nlg1 in microwells to induce presynaptic differentiation in contacting axons 49 , but this technique used platforms with a diameter of 30 μm, far from the physiological size of a synapse, and its use with most high-resolution microscopy techniques is limited. Microfluidic local perfusion chambers containing two separate cell populations were also used for the visualization and manipulation of synapses 50 . However, in that technique, endogenous synapses still formed randomly in a 1-mm-long microfluidic channel. In comparison with these studies, our system has the advantage of isolating synaptogenic processes related to one type of adhesion complex using specific coating, and to spatially control synapse formation at a micron-scale resolution. Regarding statistical yield, our technique compares favourably with the previously reported systems ( Fig. 8 ). 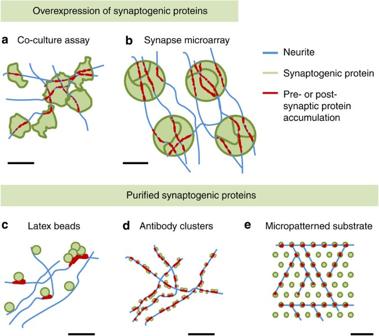Figure 8: Comparison of the various biomimetic systems used to induce synapse formation. (a) In co-culture assays, non-neuronal cells (8–17 μm in diameter) expressing synaptogenic proteins are plated on top of 1-week-old primary neuronal cultures, and the co-culture is maintained for 24–48 h. Contacting neurites form hemisynaptic puncta onto the randomly distributed heterologous cells. Because of the high variability in synaptic cluster size and the difficulty to distinguish individual clusters, the level of synapse formation is usually quantified as the global immunofluorescence intensity of synaptic staining per heterologous cell (n=20–120 cells per condition). Scale bar, 10 μm. (b) The synapse microarray is based on the co-culture system, but as non-neuronal cells are plated in an array of microwells, data collection is faster, leading to improved statistics (n>200 cells). However, the temporal resolution stays limited to 24–48 h, and synaptic contacts originating from different contacting neurites still form randomly within a 30-μm-diameter well containing the heterologous cells. Scale bar, 20 μm. (c) Synaptogenesis can also be induced by microspheres coated with purified synaptogenic proteins. The temporal resolution, corresponding to the time needed for beads to bind to neurons, is improved to 1–2 h. However, this technique is impaired by low statistics (3–15 beads bound per neuron, 10–20 cells per condition), bead aggregation and limited coverage of the beads with adhesion molecules (<30% of beads show significant recruitment of synaptic proteins). Scale bar, 10 μm. (d) Another assay consists in incubating neurons with purified proteins cross-linked by secondary antibodies, inducing the formation of individual micron-scale clusters containing counter receptors and synaptic markers within 30 min–1 h. Cross-linked adhesion molecules provide much better statistics (100–300 clusters per cell, 10–30 cells) and induce more robust recruitment of synaptic proteins, but as for beads and co-cultures, hemisynapses are still randomly distributed on the cell surface. Scale bar, 10 μm. (e) On micropatterned substrates, purified proteins are bound to ~2 μm dots arranged in a regular array, thus providing perfect spatial control, isolation of synaptic development, fairly uniform recruitment levels and large statistics production (100–400 dots per cell, 5–40 cells per condition). Synapse formation can be observed in the course of several hours; thus, the temporal resolution lies between that of co-cultures and microspheres/clusters assays. Scale bar, 10 μm. Figure 8: Comparison of the various biomimetic systems used to induce synapse formation. ( a ) In co-culture assays, non-neuronal cells (8–17 μm in diameter) expressing synaptogenic proteins are plated on top of 1-week-old primary neuronal cultures, and the co-culture is maintained for 24–48 h. Contacting neurites form hemisynaptic puncta onto the randomly distributed heterologous cells. Because of the high variability in synaptic cluster size and the difficulty to distinguish individual clusters, the level of synapse formation is usually quantified as the global immunofluorescence intensity of synaptic staining per heterologous cell ( n =20–120 cells per condition). Scale bar, 10 μm. ( b ) The synapse microarray is based on the co-culture system, but as non-neuronal cells are plated in an array of microwells, data collection is faster, leading to improved statistics ( n >200 cells). However, the temporal resolution stays limited to 24–48 h, and synaptic contacts originating from different contacting neurites still form randomly within a 30-μm-diameter well containing the heterologous cells. Scale bar, 20 μm. ( c ) Synaptogenesis can also be induced by microspheres coated with purified synaptogenic proteins. The temporal resolution, corresponding to the time needed for beads to bind to neurons, is improved to 1–2 h. However, this technique is impaired by low statistics (3–15 beads bound per neuron, 10–20 cells per condition), bead aggregation and limited coverage of the beads with adhesion molecules (<30% of beads show significant recruitment of synaptic proteins). Scale bar, 10 μm. ( d ) Another assay consists in incubating neurons with purified proteins cross-linked by secondary antibodies, inducing the formation of individual micron-scale clusters containing counter receptors and synaptic markers within 30 min–1 h. Cross-linked adhesion molecules provide much better statistics (100–300 clusters per cell, 10–30 cells) and induce more robust recruitment of synaptic proteins, but as for beads and co-cultures, hemisynapses are still randomly distributed on the cell surface. Scale bar, 10 μm. ( e ) On micropatterned substrates, purified proteins are bound to ~2 μm dots arranged in a regular array, thus providing perfect spatial control, isolation of synaptic development, fairly uniform recruitment levels and large statistics production (100–400 dots per cell, 5–40 cells per condition). Synapse formation can be observed in the course of several hours; thus, the temporal resolution lies between that of co-cultures and microspheres/clusters assays. Scale bar, 10 μm. Full size image By varying ligand coating and transfection of the corresponding receptor in neurons, this assay can easily be adapted to the study of different synaptic complexes. Although we focused here on Nlg1-dependent postsynaptic development, Nrx1β-coated micropatterned substrates are also suitable for the study of postsynaptic differentiation mediated by LRRTMs, as these adhesion molecules also bind Nrxs and interact with PSD-95 and AMPARs [51] , [52] , [53] . Inversely, micropatterns coated with LRRTMs could be used to study presynaptic assembly, as was done here with SynCAM1. Interestingly, Nrxs and Nlgs exist as many isoforms and splice variants, and their precise associations contribute to specify synapses [54] , [55] , [56] . Coating with specific α- or β-Nrx splice variants and/or neuronal transfection with the corresponding Nlg isoforms may enable the selective study of inhibitory versus excitatory synapse formation. For example, expression of Nlg2 in neurons plated on Nrx-coated substrates should favour inhibitory synapse formation [9] , [10] , [16] . Finally, as pathological mutations in Nrxs and Nlgs are related to autism, schizophrenia and X-linked mental retardation in humans [4] , such cell-chip assays of synaptic differentiation may allow the screening of new therapeutic targets for such disorders. Recent reports have identified histone deacetylase inhibitors as agents that can promote excitatory synapse maturation [49] , [57] . Our assay could be easily combined with automatized high-throughput screening systems to find such pharmacological agents, selective of pre- or postsynaptic development, and of the type of adhesion complex involved in synaptogenesis. Constructs and purified proteins Nlg1-HA, Nlg1-6His and Nrx1β-Fc plasmids were generous gifts from P. Scheiffele (Biozentrum, Basel). Nrx1β-HA was a gift from M. Missler (Münster University). SynCAM1-Fc was a gift from T. Biederer (Yale University). PSD-95 with a C-terminal GFP or mCherry tags were previously reported 15 . The production of Nrx1β-Fc and SynCAM1-Fc proteins, and the purification on G protein columns was previously described [12] , [40] . Nlg1-6His was produced following the same protocols, purified on a Ni-Sepharose column (His Trap HP; GE Healthcare) and eluted using 500 mM imidazole. The imidazole buffer was exchanged with PBS by dialysis. Recombinant N-cadherin-Fc was purchased from R&D Systems as a 100 μg ml −1 solution. Micropatterned substrates Micropatterned substrates were obtained from CYTOO ( www.cytoo.com ) as a custom designed ‘Ready to Coat’ product (ref 10-950-00), made according to a previously published protocol 58 . Specifically, hydrophilic dots of 1.5 μm diameter were separated by 5 μm, and were surrounded by a uniform cytophobic environment made of polyethyleneglycol. Substrates were then treated with 40 μg ml −1 polylysine (Sigma), which adsorbed to the hydrophilic dots, dried and stored at 4 °C. One day before plating cells, a 9:1 ratio of unlabelled and Cy5-conjugated goat anti-human Fc antibodies (Jackson Immunoresearch) or Cy5-conjugated rabbit anti-6His antibodies (Santa Cruz) were diluted at 0.023 mg ml −1 in borate buffer (boric acid 0.2 M, pH 8.5) and were centrifuged for 10 min at 14,000 r.p.m. and 4 °C. Micropatterned substrates were flipped onto a 200-μl drop of the antibody mixture on parafilm previously sterilized with ultraviolet radiation, and incubated at room temperature for 4–5 h. Substrates were then washed with borate buffer and were incubated overnight at 4 °C with purified Nrx1β-Fc, SynCAM1-Fc, N-cadherin-Fc or Nlg1-6His (0.04 mg ml −1 in boric acid, previously centrifuged for 10 min at 14,000 r.p.m.). Substrates were placed into six-well plates, washed with borate buffer and left with MEM containing 10% horse serum for 1–2 h in the incubator (37 °C, 5% CO 2 ). Cell culture and transfection Dissociated hippocampal neurons from E18 rat embryos were plated on the substrates (100,000 cells per coverslip). Four to five hours after plating, substrates were carefully washed with neurobasal medium (NB) supplemented with B27 (37 °C) to remove unattached cells, and the medium was replaced with conditioned NB medium (NB+B27 medium previously incubated for 4 days in dishes containing a glial cell layer). Neurons were transfected at DIV 3 using Effectene (Qiagen), according to the manufacturer’s instructions, using 1 μg total DNA per micropatterned coverslip. For cotransfections of Nlg1 and PSD-95:EGFP, or Nlg1 and EGFP, a 2:1 DNA ratio was used. All institutional guidelines on animal welfare were followed. Immunocytochemistry Neuronal cultures were fixed for 10 min in warm 4% paraformaldehyde–4% sucrose in PBS, and the remaining active sites were saturated with 50 mM NH 4 Cl in PBS for 15 min. Non-specific binding was blocked with PBS containing 1% BSA. To visualize Nlg1 at the neuronal surface, neurons transfected with Nlg1-HA were stained using rat anti-HA (Roche; 1:400) followed by Alexa568-conjugated goat anti-rat antibody (2 mg ml −1 ; Invitrogen; 1:800) for 30 min at room temperature. To stain endogenous PSD-95, synapsin, SynCAM1 or N-cadherin, cultures were fixed and permeabilized with 0.1% Triton X-100 in PBS for 5 min, then labelled for 1 h with 1:400 dilutions of mouse anti-PSD-95 (Neuromab), mouse anti-synapsin (Synaptic Systems), mouse anti-N-cadherin (BD Transduction Labs) or rabbit anti-SynCAM1 (Abcam), followed by Alexa568-conjugated goat anti-mouse or anti-rabbit antibodies, respectively (2 mg ml −1 ; Molecular Probes; 1:800). To stain endogenous AMPARs, a 10-min live surface labelling was performed at 37 °C with a 1:100 dilution of a monoclonal anti-GluA2 antibody (a gift of E. Gouaux, Vollum Institute, Portland) in culture medium, followed by fixation and BSA blocking. Staining was revealed using Alexa568-conjugated goat anti-mouse antibody (2 mg ml −1 ; Invitrogen; 1:800). To localize active presynapses, cells were labelled for 10 min using a 1:100 dilution of anti-synaptotagmin1 lumenal domain conjugated to Oyster 550 fluorophore (Synaptic Systems) in observation medium, then fixed as described above. Coverslips were mounted in Mowiol (Calbiochem). Image analysis Immunostainings were visualized on a Leica DM R upright epifluorescence microscope (Leica Microsystems, Wetzlar, Germany) equipped with a × 63/1.32 numerical aperture (NA) objective and appropriate filter sets from Chroma (GFP: excitation S490/20 nm, dichroic 86100bs, emission S528/38 nm; TRITC (tetramethylrhodamine-5-(and-6)-isothiocyanate (5(6)): excitation S555/28 nm, dichroic 101848, emission S617/73; Cy5: excitation S635/20, dichroic 101848, emission S685/40 nm). Images were acquired with a charge-coupled device (CCD) camera (HQ CoolSnap; Roper Scientific, Evry, France), using the Metamorph software (Universal Imaging Corp.). The enrichment factors of Nlg1 and PSD-95 at the patterns were measured on three randomly chosen dendritic areas of each neuron and were calculated using an automatic programme written in Metamorph. Briefly, the outlines of the corresponding patterns were transferred to the Nlg1 and PSD-95 image, where the outline of the neurite was determined by a threshold function ( Supplementary Fig. S1 ). The patterns that did not overlap with the threshold area were eliminated from further quantification. An enrichment index was calculated by dividing the fluorescence intensity within each dot for the thresholded area, by the average intensity measured from dendritic parts located outside patterns. Detection of synapsin or PSD-95 clusters and quantification of their overlapping area with micropatterns was carried out using a custom-developed plugin for Image J (NIH) described previously [15] . Briefly, synapsin or PSD-95 signals of axonal or dendritic segments, respectively, and Cy5 signals corresponding to micropatterns were separately segmented. The overlapping area of synaptic and micropattern signals was then calculated on the overlaid image, and the percentage of synapsin or PSD-95 signal overlapping more than 50% with a micropattern was determined and averaged on a per cell basis ( Supplementary Fig. S6 ). The value for a random distribution of puncta was calculated as the fractional area of micropatterns occupying the field of view. Live cell imaging Primary hippocampal neurons (DIV 7) growing on Nrx1β-Fc-coated micropatterned substrates and expressing Nlg1 and PSD-95:EGFP were mounted on an open chamber containing a 1:1 mixture of Tyrode solution and conditioned NB medium. Cells were then observed on an inverted Leica DMI 6000 microscope (Leica Microsystems), equipped with a CCD camera (CoolSnap HQ2; Roper Scientific) and a thermostatic box (Life Imaging Services, Basel, Switzerland) providing 37 °C and 5% CO 2 . Long-term acquisitions were made by using a HCX PL APO CS × 63 oil 1.32 NA objective and illumination with a mercury lamp and appropriate excitation/emission filters from Chroma (GFP: excitation HQ 480/30 nm, dichroic 86100bs, emission S528/38 nm; Cy5: excitation HQ630/20 nm, dichroic 101848, emission S685/40 nm). PSD-95:EGFP images were recorded every 10 min for 5 h, whereas Cy5 images of the pattern were taken only twice, one before and one after the acquisition. For determination of the growth and stage of differentiation of neurons cultured on micropatterned substrates with different coatings (Nrx1β-Fc, N-cadherin-Fc and PLL), time-lapse imaging of neurons at DIV 1–2 was carried out using a × 40 phase-contrast objective on a Biostation machine equipped with a 5% CO 2 air flow and stable temperature control (a kind loan of Nikon, France). Images were analysed using the NeuroJ plugin (NIH). Glutamate uncaging Primary hippocampal neurons (DIV 7–8) growing on Nrx1β-Fc-coated micropatterned substrates and transfected with PSD-95:mCherry and Nlg1 were loaded with 2.5 μM Fluo-4-AM (Invitrogen) for 5 min in culture medium, then mounted in Tyrode (30 mM glucose, 120 mM NaCl, 5 mM KCl, 0.1 mM MgCl 2 , 2 mM CaCl 2 and 25 mM HEPES), supplemented with 5 mM MNI-glu (Tocris), and 1 μM tetrodotoxin to prevent action potentials. The observation chamber was placed on a confocal scanning laser microscope (TCS SP5; Leica) thermostated to 37 °C and equipped with a pulsed bi-photon laser (Mai Tai; Spectra-Physics) tuned to 750 nm. For the fluorescence recordings, a fivefold zoomed area of 256 × 256 pixels was scanned at 700 Hz by the 488-nm Argon laser line, and the fluorescence light between 500 and 530 nm was collected by a photomultiplier, using a HCX PL APO CS × 63/1.32 NA oil objective and a pinhole open to three times the Airy disk (180 μm). After recording a baseline, one 10 ms pulse of bi-photon light restricted to a small region of interest (~7 μm 2 ) was given to uncage MNI-glu. Fluorescence signals were then recorded every 200 ms for 1 min. To quantify the calcium responses, the Fluo-4 intensity values at given locations were normalized to the average fluorescence intensity before the bi-photon light pulse. When MNI-glu was omitted, no calcium transient was observed. In some experiments, MNI-glu was uncaged in the vicinity of synapses in 3-week-old neurons transfected with Homer-DsRed and growing on regular glass coverslips. Mosaic reconstruction Individual high-magnification images were taken using a HCX PL APO CS × 63 oil 1.32 NA objective on the microscope described above for live cell recordings (Leica DMI 6000), using the Scan slide module of MetaMorph, which drives a motorized stage Scan IM (Märzhäuser, Wetzlar, Germany). Mosaic images were then created from 20–30 individual images using a stitching function. Single-molecule tracking of AMPARs Primary hippocampal neurons (DIV 7–8) growing on either Nrx1β-Fc- or Fc-coated micropatterned substrates, and coexpressing Nlg1 and Homer1c:GFP, were mounted in Tyrode in an open observation chamber (Life Imaging Services). The chamber was placed on an inverted microscope (Nikon Ti-E Eclipse) equipped with an electron multiplying CCD camera (Evolve, Roper Scientific), a thermostatic box (Life Imaging Services) providing air at 37 °C, and an APO total internal reflection fluorescence microscope × 100 oil 1.49 NA objective. The lateral movement of individual AMPARs was followed by single-molecule tracking 30 . Monoclonal anti-GluA2 antibodies were conjugated with ATTO 647N dyes (Attotec) according to the manufacturer’s protocol. Surface AMPARs were continuously and stochastically labelled in solution, with a 1:6,000 dilution of ATTO647N-conjugated anti-GluA2 antibodies. The samples were imaged by oblique illumination performed with the 633-nm line of a HeNe laser (Roper Scientific) and dichroic mirror (Di01-R635; SemRock), allowing the excitation of individual ATTO-647N molecules, which are bound to the cell surface, without illuminating the molecules in the solution above. Fluorescence was collected using a 676/29-nm emission filter (SemRock) placed on a filter wheel (Suter). Five stacks of 4,000 consecutive frames were obtained from each cell, with an integration time of 50 ms. Detection of single molecules and the analysis of image stacks were processed using a custom programme running on Metamorph software (Molecular Devices) described earlier 59 . This programme allows the identification of each dye as individual objects, by fitting a two-dimensional Gaussian to the intensity patterns of its fluorescent signal (spots), and connects successive positions. The instantaneous diffusion coefficient, D , was calculated for each trajectory, from linear fits of the first four points of the mean square displacement function versus time. How to cite this article: Czöndör, K. et al . Micropatterned substrates coated with neuronal adhesion molecules for high-content study of synapse formation. Nat. Commun. 4:2252 doi: 10.1038/ncomms3252 (2013).